Giant magnetostriction in annealed Co1−xFexthin-films Chemical and structural heterogeneity and the resulting interaction of coexisting phases can lead to extraordinary behaviours in oxides, as observed in piezoelectric materials at morphotropic phase boundaries and relaxor ferroelectrics. However, such phenomena are rare in metallic alloys. Here we show that, by tuning the presence of structural heterogeneity in textured Co 1−x Fe x thin films, effective magnetostriction λ eff as large as 260 p.p.m. can be achieved at low-saturation field of ~10 mT. Assuming λ 100 is the dominant component, this number translates to an upper limit of magnetostriction of λ 100 ≈5 λ eff >1,000 p.p.m. Microstructural analyses of Co 1−x Fe x films indicate that maximal magnetostriction occurs at compositions near the (fcc+bcc)/bcc phase boundary and originates from precipitation of an equilibrium Co-rich fcc phase embedded in a Fe-rich bcc matrix. The results indicate that the recently proposed heterogeneous magnetostriction mechanism can be used to guide exploration of compounds with unusual magnetoelastic properties. Magnetostrictive thin films are at the heart of many microsystem applications, especially in microelectromechanical systems as powerful transducers for microactuators [1] , [2] , [3] . Their major advantages over other smart materials include remote control operation, simple actuator designs, and compatibility with semiconductor manufacturing processes that facilitates integration in current microelectronic technologies [4] , [5] , [6] , [7] , [8] . To fully exploit their capabilities and meet the stringent needs of microactuator and sensor applications, small driving magnetic fields on the order of mT are desirable. Interest in magnetostrictive films began in the mid-1970s [9] , and various single layer and multilayer magnetostrictive films exhibiting large magnetostriction have been reported to date [2] , [3] , [5] , [10] , [11] , [12] , [13] , [14] , [15] , [16] . Among them, rare-earth–Fe-alloy thin films show the largest magnetostriction including Tb–Dy–Fe films that can generate strains over 1,000 p.p.m. in polycrystalline thin films. (In bulk single crystals, Tb 0.3 Dy 0.7 Fe 2 can exhibit magnetostriction 3/2 λ 111 as large as 2,600 p.p.m.) Despite the giant magnetostriction, their large magnetocrystalline anisotropy that results in a high-saturation field (H>0.1 T) has generally restricted their use in practical applications, thereby spurring the inquiry into alternative new materials. It is also increasingly important to find rare-earth free compounds from the cost and availability points of view. Recently, Fe 1−x Ga x alloys have generated significant research interest owing to their large magnetostriction. It was found that alloying Fe with 20 at.% Ga in single crystal Fe 1−x Ga x alloys yields a large magnetostrictive tetragonal strain of 3/2 λ 100 ≥400 p.p.m., where λ 100 is the magnetostriction coefficient with the field applied in the [100] crystallographic direction of the sample [17] . Moreover, these alloys show good mechanical properties at low fields [18] . These characteristics have made the Fe–Ga alloys attractive alternatives to existing rare-earth-based magnetostrictive materials. One of the striking features about the Fe 0.8 Ga 0.2 alloy is the phase dynamics under which enhancement in magnetostriction occurs: a disordered body-centred-cubic (bcc) α-Fe (or A2) phase is in metastable equilibrium with a D0 3 (ordered bcc) phase [19] . A proposed model for Fe 1−x Ga x suggests that the D0 3 nanoclusters embedded in the A2 matrix give rise to a magnetic field induced rotation leading to the large magnetostriction [20] , [21] . Also, in the previously studied Fe–Al alloy system, a significant increase in magnetostriction was observed in compositions at the D0 3 /A2-phase boundary. An emerging trend is that magnetostriction enhancement in Fe-based systems occurs for compositions near structural phase boundaries. An analogy with giant electrostriction of ferroelectric solid solution and relaxors [22] , [23] also points to the intriguing possibility that some structural boundaries in magnetic materials can act as property-enhancing morphotropic-phase boundaries. Indeed, Yang et al . have reported a rhombohedral/tetragonal morphotropic phase boundary with enhanced magnetostrictive properties in the TbCo 2 –DyCo 2 system occurring below 160 K (ref. 24 ). It is of fundamental interest to identify new alloys with large magnetostriction and to help understand the origin of magnetostriction enhancement. Here we investigated the Co–Fe system with a focus on the (fcc+bcc)/bcc phase boundary around the Co 0.75 Fe 0.25 composition. The bulk Co–Fe-phase diagrams [25] , [26] shows that the α-Fe bcc phase exists at higher temperatures for all compositions. At temperatures lower than 912 °C and Co concentrations >50 at.%, the bcc phase intersects with a mixed phase region of face-centred-cubic (fcc) Co and bcc Fe phases. Applying the scenario described above for the Fe 0.8 Ga 0.2 alloy, it is at this (fcc+bcc)/bcc boundary that the enhancement of the magnetostriction would be expected to occur. Early studies performed on bulk Co–Fe alloys showed two peaks in the magnetostriction versus composition curve: one at the Co 0.7 Fe 0.3 and the other near the equiatomic compositions of Co 0.5 Fe 0.5 , yielding magnetostrictions of 90 p.p.m. and 75 p.p.m., respectively [27] , [28] . In later experiments, Hall reported magnetostriction of λ 100 ~150 p.p.m. for annealed bulk single crystal Fe 0.5 Co 0.5 alloys [29] , [30] . Since then, several studies on alloys of the 50:50 composition in bulk [31] , [32] and thin films [10] , [11] , [13] , [33] have been reported, but little attention has been given to the other compositions in the phase diagram. In a recent bulk experiment, magnetostriction of 150 p.p.m. was observed in a homogenized arc-melted Co 0.7 Fe 0.3 alloy, which was annealed at 800 °C (ref. 34 ). In this study, we investigate the composition and thermal process-dependent magnetostrictive and microstructural properties of Co 1−x Fe x alloy thin films, prepared using a co-sputtering-based composition-spread approach [16] , [35] , [36] , [37] . This technique facilitates synthesis and screening of large compositional landscapes in individual studies and allows rapid identification of compositions with enhanced physical properties. We find that depending on the processing conditions, large magnetostriction is obtained at different compositions. Correlation with microstructural properties of the films clearly shows that magnetostriction enhancement is observed at the (fcc+bcc)/bcc phase boundary. This behaviour is similar to the occurrence of large magnetostriction in Fe 1−x Ga x alloys and can be explained using the heterogeneous magnetostriction model [20] , [21] . Cantilever measurements Magnetostriction measurements were performed at room temperature on arrays of Si/SiO 2 micro-machined cantilevers, on which 0.5-μm±0.01-μm thick composition gradient Co 1−x Fe x (0.1≤x≤ 0.9) films were sputter-deposited: one in the as-deposited state, and two after thermal treatments; one which was annealed for 1 h at 800 °C and slow-cooled, and the other which was annealed for 1 h at 800 °C and water-quenched. 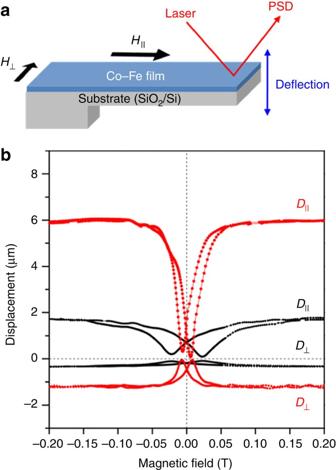Figure 1: Technique for determining thin film magnetostriction. (a) Schematic showing the two field directions which were applied in the plane of the cantilever samples, (b) plot of the displacement (μm) versus magnetic field for an as-deposited (black curves) and an annealed and quenched (red curves) Co0.66Fe0.34sample.D||andD⊥indicate the displacements obtained from magnetic fields applied parallel (H∥) and perpendicular (H⊥) in the plane of the cantilever samples as shown in (a). PSD, position sensitive detector. Figure 1a shows the two field directions that were applied in the plane of the cantilever samples (for details, see Methods ). Displacement measurements were recorded for magnetic fields applied parallel and perpendicular to the length of the cantilever, but always parallel to film plane. Figure 1b shows a plot of the displacement (μm) versus magnetic field for an as-deposited and a quenched Co 0.66 Fe 0.34 sample. Figure 1: Technique for determining thin film magnetostriction. ( a ) Schematic showing the two field directions which were applied in the plane of the cantilever samples, ( b ) plot of the displacement (μm) versus magnetic field for an as-deposited (black curves) and an annealed and quenched (red curves) Co 0.66 Fe 0.34 sample. D || and D ⊥ indicate the displacements obtained from magnetic fields applied parallel ( H ∥ ) and perpendicular ( H ⊥ ) in the plane of the cantilever samples as shown in ( a ). PSD, position sensitive detector. 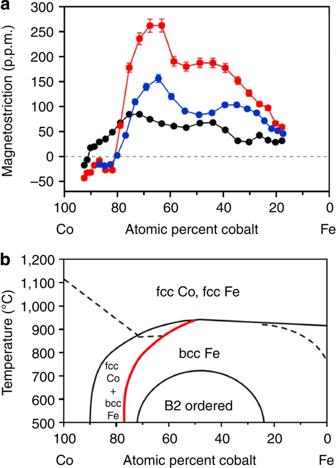Figure 2: Magnetostriction in Co1−xFexfilms and corresponding Co–Fe-phase diagram. (a) Magnetostriction variation versus atomic percent cobalt for three differently prepared Co1−xFexcomposition spreads, as-deposited (black dots), slow-cooled (blue dots), quenched (red dots), (b) Co–Fe-phase diagram. The error bars in (a) are calculated from the uncertainty in Young's modulus and the standard deviation in cantilever displacement due to magnetostriction. The red curve highlights the approximate phase boundary between (fcc Co + bcc Fe) and bcc Fe. Full size image Figure 2a shows the measured effective magnetostriction as a function of atomic composition for three composition spread films: as-deposited state (black circles), annealed and slow-cooled (blue circles), and annealed and water-quenched (red circles). The room temperature as-deposited composition spread shows that as Co is substituted for Fe, two composition regions with enhanced magnetostriction appears. The first enhanced region is centred around the well-studied Co 0.5 Fe 0.5 composition and reaches a maximum magnetostriction of 67±5 p.p.m. at Co 0.44 Fe 0.56 , whereas the maximum value of the second enhanced region is 84±5 p.p.m. near Co 0.73 Fe 0.27 , in the vicinity of the phase boundary of (fcc+bcc)/bcc of the Co–Fe-phase diagram shown in Figure 2b . This composition trend is similar to the one reported for bulk materials where two peaks of magnetostriction were observed near the Co 0.5 Fe 0.5 and Co 0.7 Fe 0.3 compositions [27] , [28] . The magnetostriction value of 67 p.p.m. obtained for our Co 0.5 Fe 0.5 films is in good agreement with previous polycrystalline thin film [10] and bulk [38] reports. Figure 2: Magnetostriction in Co 1−x Fe x films and corresponding Co–Fe-phase diagram. ( a ) Magnetostriction variation versus atomic percent cobalt for three differently prepared Co 1−x Fe x composition spreads, as-deposited (black dots), slow-cooled (blue dots), quenched (red dots), ( b ) Co–Fe-phase diagram. The error bars in ( a ) are calculated from the uncertainty in Young's modulus and the standard deviation in cantilever displacement due to magnetostriction. The red curve highlights the approximate phase boundary between (fcc Co + bcc Fe) and bcc Fe. Full size image The annealed and slow-cooled spread (blue circles) shows significant increases in magnetostriction over the majority of the composition range studied here, and the two broad peaks of magnetostriction, observed in the as-deposited sample, have now shifted to lower Co content by ~7 at.%. The maximum magnetostrictions are now 103±6 and 156±7 p.p.m. for compositions of Co 0.4 Fe 0.6 and Co 0.66 Fe 0.34 , respectively, in the slow-cooled spread. Annealing and quenching the spreads (red circles) leads to an even larger enhancement in magnetostriction over a large composition range. There are two noticeable features about this heat treatment. First, starting from about Co 0.18 Fe 0.82 , as more Co is substituted for Fe, the magnetostriction increases steadily up to 180 p.p.m., and a broad plateau is observed in magnetostriction for compositions between 38 and 56 at.% Co. On further increase in Co content, the magnetostriction value rises to an unusually high level between 60 and 75 at.% Co, with a maximum magnetostriction of 260±10 p.p.m. at the Co 0.66 Fe 0.34 composition. Beyond Co 0.75 Fe 0.25 , the magnetostriction drops precipitously as more Co is added and becomes negative at compositions >82 at.% Co. At this (Co 0.66 Fe 0.34 ) composition, the magnetostriction of the annealed and water-quenched sample is more than three times the as-deposited value. Two repeat experiments with the same thermal processing have resulted in the same magnetostriction values across the spread. We have confirmed, using wavelength dispersive X-ray spectroscopy, that the composition distribution across the spread remains unchanged after thermal treatment. Synchrotron micro-diffraction investigation To explore the structural origin of this enhancement in magnetostriction, synchrotron X-ray micro-diffraction was carried out on the three composition spreads to map their phase distribution. 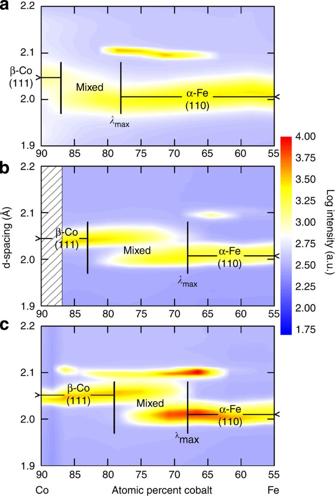Figure 3: Synchrotron microdiffraction of Co1−xFexthin films. Intensity plots of (a) as-deposited, (b) annealed and slow-cooled, (c) annealed and water-quenched composition spread samples. The diffracted intensity is presented in colour code to the right of the figure. The black line markedλmaxin each spread indicates the approximate composition of the (fcc+bcc)/bcc phase boundary. This also corresponds to the compositions of maximum magnetostriction presented inFigure 2a. No data was collected in the hatched region of (b). Figure 3 shows density plots of the measured d-spacings as a function of atomic composition for the (a) as-deposited, (b) annealed and slow-cooled, and (c) annealed and water-quenched samples. In Figure 3a (as-deposited spread), a dominant α-Fe (110) phase spans almost the entire Co–Fe composition range studied here. The bcc phase is maintained to compositions with Co concentration as high as 90%. However, near 78 at.% Co, a weak reflection between d ~2.05 and d ~2.10 Å, corresponding to fcc (111) reflection of fcc β-Co begins to appear. These two phases coexist (mixed phase) over ~7 at.% as indicated in the figure. Note that the composition, where the β-Co (111) peak first appears (Co 78 at.%), is coincident with the composition that shows the largest magnetostriction in the as-deposited film ( Fig. 2a ). Figure 3: Synchrotron microdiffraction of Co 1−x Fe x thin films. Intensity plots of ( a ) as-deposited, ( b ) annealed and slow-cooled, ( c ) annealed and water-quenched composition spread samples. The diffracted intensity is presented in colour code to the right of the figure. The black line marked λ max in each spread indicates the approximate composition of the (fcc+bcc)/bcc phase boundary. This also corresponds to the compositions of maximum magnetostriction presented in Figure 2a . No data was collected in the hatched region of ( b ). Full size image Figure 3b shows the diffraction data for the same composition spread after it was annealed at 800 °C and slow-cooled. The peak near 2.01 Å that was prominent in the as-deposited state remains, but the full-width half-maximum value for the reflection is half of the as-deposited value, indicating a well-crystallized bcc (110) phase peak. However, the most striking feature in this figure is the fcc (111) β-Co peak at d ~2.05 Å. This peak which was weak and broad in the as-deposited state has now evolved into a well-pronounced peak and extends further into the Fe-rich region (up to 30 at.% Fe). The growth of this fcc phase during the anneal has resulted in a broader composition region of two-phase mixture compared with the as-deposited state. More importantly, there is a shift in the (fcc+bcc)/bcc phase boundary to lower Co content (~Co 66 at.%), and this composition is again coincident with the composition that shows the highest magnetostriction ( Fig. 2a ). Figure 3c shows the density diffraction plot of the annealed and water-quenched composition spread samples. In structure, it mirrors the slow-cooled spread, and a well-defined (111) β-Co peak overlaps with the (110) α-Fe peak to create an fcc Co+bcc Fe-phase mixture region, and the phase boundary is shifted to ~66 at.% Co. This result closely follows the Co–Fe-phase diagram ( Fig. 2b ) in which the red line indicating the (fcc+bcc)/bcc phase boundary trends towards lower Co content as the temperature is increased. The key finding here is that, in the slow-cooled and the quenched spreads, the maximum enhancement of magnetostriction occurs at the (fcc+bcc)/bcc phase boundary that is where the fcc phase first appears. The peak seen in all the three spreads at 2.10 Å is from an oxidized thin surface layer of CoO ( T N =287 K), which does not contribute to the room temperature magnetic properties discussed here. Electron microscopy measurements To further investigate the microstructural details, two highly magnetostrictive samples (as-deposited and quenched) of Co 0.73 Fe 0.27 films were analysed by transmission electron microscopy (TEM). 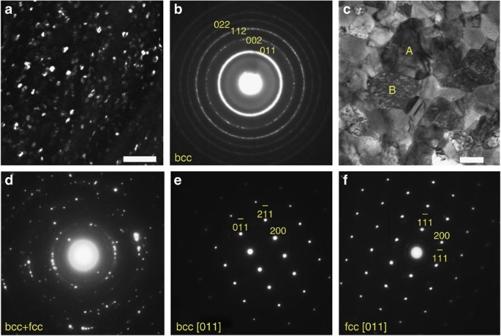Figure 4: TEM images and diffraction of a highly magnetostrictive as-deposited and an annealed Co–Fe sample. TEM images of Co0.73Fe0.27of (a) (110) dark field image of as-deposited sample, the scale bar is 50 nm. (b) corresponding SAED pattern of the as-deposited, (c) bright field image of annealed sample, the scale bar is 200 nm. (d) SAED pattern of the same sample as (c) using ~1.5-μm-diameter aperture showing the mixture structure of bcc and fcc phases, (e) [011] bcc diffraction pattern from grain marked 'A' in (c), and (f) [011] fcc diffraction pattern from grain marked 'B' in (c). Figure 4a shows a dark-field image of the (011) reflections from the selected area electron diffraction (SAED) pattern ( Fig. 4b ) of the as-deposited sample. The image shows a microstructure consisting of randomly oriented nanosized polycrystals of an average grain size of ~10 nm. The SAED pattern of Figure 4b reveals diffraction rings indicative of the random crystallographic orientations of the nanograins of the as-deposited state. All diffraction rings are identified as that of a bcc structure consistent with the synchrotron data in Figure 3a . Figure 4: TEM images and diffraction of a highly magnetostrictive as-deposited and an annealed Co–Fe sample. TEM images of Co 0.73 Fe 0.27 of ( a ) (110) dark field image of as-deposited sample, the scale bar is 50 nm. ( b ) corresponding SAED pattern of the as-deposited, ( c ) bright field image of annealed sample, the scale bar is 200 nm. ( d ) SAED pattern of the same sample as ( c ) using ~1.5-μm-diameter aperture showing the mixture structure of bcc and fcc phases, ( e ) [011] bcc diffraction pattern from grain marked 'A' in ( c ), and ( f ) [011] fcc diffraction pattern from grain marked 'B' in ( c ). Full size image Figure 4c and 4d display a bright-field image and the SAED pattern, respectively, of a sample which was water-quenched following an anneal. Compared with Figure 4a, 4c shows a much coarser structure with grain sizes up to ~100 nm. The corresponding SAED pattern taken over a large area shows that, in addition to the expected bcc reflections, a second phase (fcc) is present. Detailed SAEDs from individual grains marked A and B in Figure 4c of the annealed sample have been used to identify the two phases to be bcc ( Fig. 4e ) and fcc ( Fig. 4f ), respectively. Further analysis by energy-dispersive X-ray spectroscopy (not shown) on these grains revealed that the bcc phase is Fe-rich and the fcc phase is Co-rich, consistent with the Co–Fe-phase diagram and synchrotron results of Figures 2b and 3c , respectively. In some of the samples, the annealing had resulted in formation of a thin film/substrate interface layer of Fe–Co–Si–O (<50 nm in thickness), which is not expected to contribute to the properties observed here. To better understand the relationship between the cooling process and the magnetostriction properties, a detailed TEM analysis was performed on individual grains from both slow-cooled and water-quenched samples. 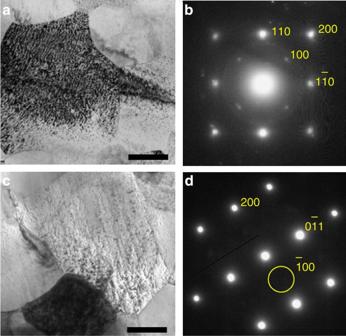Figure 5: TEM images and diffraction of a slow-cooled and a water-quenched sample. TEM image and diffraction of Co0.66Fe0.34grains from the slow-cooled (a,b) and water-quenched (c,d) samples. The bright field images (a,c) show the location of the corresponding SAED patterns (b,d). The [001] pattern from the slow-cooled grain (b) shows a typical bcc pattern with the addition of 4 dim {100} reflections that indicate B2 ordering. The absence of the {100} reflection in the [011] SAED pattern of the quenched grain indicates the grain is disordered. The scale bars in (a,c) are 200 nm. Figure 5a displays a bright field image of a bcc grain from the slow-cooled sample with a composition of Co 0.66 Fe 0.34 and a λ eff of 156 p.p.m. The four weak inner reflections in the SAED pattern of this grain, shown in Figure 5b , indicates a beam direction of [001] onto a highly ordered B2 structure. In contrast, the image and SAED pattern ( Fig. 5c,d ) of a quenched sample of the same composition whose λ eff is 260 p.p.m. shows no diffracted [100] spots and thus no evidence of ordering. This demonstrates that ordering suppresses magnetostriction and is the reason for the reduced magnetostriction observed in the slow-cooled samples as compared with the water-quenched samples. Figure 5: TEM images and diffraction of a slow-cooled and a water-quenched sample. TEM image and diffraction of Co 0.66 Fe 0.34 grains from the slow-cooled ( a , b ) and water-quenched ( c , d ) samples. The bright field images ( a , c ) show the location of the corresponding SAED patterns ( b , d ). The [001] pattern from the slow-cooled grain ( b ) shows a typical bcc pattern with the addition of 4 dim {100} reflections that indicate B2 ordering. The absence of the {100} reflection in the [011] SAED pattern of the quenched grain indicates the grain is disordered. The scale bars in ( a , c ) are 200 nm. Full size image The substantial enhancement of magnetostriction in annealed Co 1−x Fe x thin film alloys observed here, particularly in the water-quenched samples, underscores the dependence of the microstructure on processing and its close ties with magnetostriction. It is remarkable that annealing the sample at a temperature/composition close to the (fcc+bcc)/bcc phase boundary followed by quenching would yield magnetostriction values more than three times that of its as-deposited state. In Figure 2a , we see that the peak of magnetostriction shifts ~7 at.% to Co lower composition after annealing. Similarly, the (fcc+bcc)/bcc phase boundary in Figure 3 shifts by about the same amount in the annealed spreads indicating that the peak of magnetostriction is linked to this phase interface. From Figure 3 , we also see that the dominant phase at the (fcc+bcc)/bcc boundary is bcc. The TEM data from Figure 4c,d of an annealed sample also confirms that the composition consists of the predominant bcc phase and a secondary fcc phase. As discussed above, precipitation of the fcc Co-rich grains into the bcc α-Fe matrix is the cause of the increase in magnetostriction observed in the annealed samples. This is analogous to the Fe–Ga alloy system where the maximum magnetostriction is observed near the A2/D0 3 phase boundary at the composition of Fe 0.8 Ga 0.2 (ref. 39 ). In a recent report, a significant amount of D0 3 nanoprecipitates dispersed in the host A2 matrix was observed in Fe–Ga samples, and the D0 3 nanoprecipitates are believed to have a significant role in the enhancement of the magnetostriction [40] . The interpretation is that coarsening resistant metastable martensitic clusters form, when D0 3 precipitates equilibrate by undergoing a displacive transition and it is these martensitic clusters that lead to magnetostriction. It is likely that the Co-rich precipitates in our Co–Fe films function in much the same way as the D0 3 precipitates in the Fe–Ga alloys. There is a strong dependency of the magnetostriction on the cooling process in the present Co–Fe alloys. According to the Co–Fe-phase diagram [25] , the B2 phase exists in the composition region between 28 and 78 at.% Fe. When slow-cooled, samples in this composition space are expected to enter the B2 phase and become ordered as illustrated in Figure 5 , and there is a substantial difference in magnetostriction of the slow-cooled (B2-ordered) and water-quenched (disordered) samples. Similar ordering dynamics was observed in Fe–Ga where a disordered solid solution is the preferred phase for achieving large magnetostriction [39] , [41] . In the case of Fe 0.8 Ga 0.2 , martensitically transformed precipitates would act as tetragonal defects embedded in the matrix [20] , [21] . Their orientations can be rotated by applying an external stress or a magnetic field. The magnitude of the resulting magnetostrictive strains is dependent on the density of the precipitates in the matrix. In our Co–Fe films, a similar scenario can be envisioned at the (fcc+bcc)/bcc matrix boundary. The displacive transition would be bcc to fct (fcc). It is possible that the bcc phase consists of coherently stabilized D0 3 (ref. 42 ). It is the reorientation of the tetragonal precipitates due to magnetic field that would give rise to the magnetostriction observed here. From other TEM micrographs obtained from the quenched Co 0.66 Fe 0.34 , we estimate the volume fraction of the fcc precipitates to be ~3.4×10 −3 . Multiplying this with the un-relaxed bcc/fcc Bain strain of 0.30, which translates to magnetostriction on reorientation, we arrive at an upper limit magnetostriction value of 1,400×10 −6 . As our annealed films are textured, the relationship of the effective magnetostriction to the cubic constants is given by [43] : If we assume that the reorientation strain dominates, that is, λ 111 ≪ λ 100 , then Thus, with a simple heterogeneous mixture model, we can obtain qualitative agreement between the observed value of magnetostriction and the expected value from reorientation of the precipitates. We also observe significant reduction in the coercive field as well as rounding of the M–H curves on annealing and quenching of the film ( Fig. 6 ). Compared with the as-deposited film, the quenched film displays a much smaller coercive field of ~5 mT. This is consistent with the heterogeneous magnetostriction model that an applied field leads to reconfigurations of fct microdomains and the bcc magnetic domains resulting in reduction of the coercive field. Additionally, we see a drop in Young's modulus at the onset of magnetostriction enhancement as a function of composition in the quenched sample as predicted in the model, see Figure 7 . 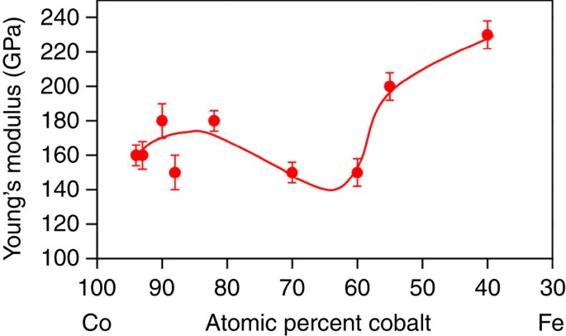Figure 7: Dependence of Young's modulus on Co composition for annealed samples. There is a decrease or 'softening' of the elastic properties in the vicinity of large magnetostriction. 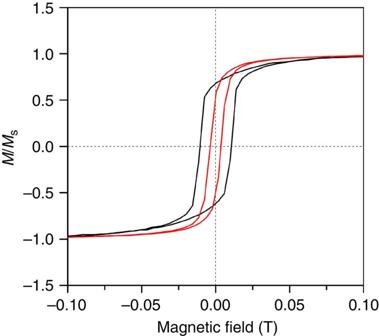These observations together provide strong evidence that the proposed precipitate magnetostriction model for Fe–Ga maybe at work here in the water-quenched Co–Fe films at the (fcc+bcc)/bcc structural boundary. Figure 6: In-plane magnetization versus field curves for as deposited and quenched Co0.66Fe0.34films. The black plot is the as-deposited and the red plot is for the annealed and water-quenched sample. The quenched sample shows a much reduced coercive field. Figure 6: In-plane magnetization versus field curves for as deposited and quenched Co 0.66 Fe 0.34 films. The black plot is the as-deposited and the red plot is for the annealed and water-quenched sample. The quenched sample shows a much reduced coercive field. Full size image Figure 7: Dependence of Young's modulus on Co composition for annealed samples. There is a decrease or 'softening' of the elastic properties in the vicinity of large magnetostriction. Full size image The low-field room-temperature magnetostriction reported here is among the highest for a rare-earth-free alloy and is promising for micro-actuator applications. A larger implication of the observed enhancement at the phase boundary and the striking qualitative agreement between the overall properties of the quenched films and the predictions of heterogeneous magnetostriction is that the model can perhaps be extended as a guideline to explore compositions with enhanced magnetoelastic properties in other material systems. Growth and annealing of the composition spread thin films Thin film Co 1−x Fe x binary composition spreads (thickness 0.5 μm±0.01 μm) were deposited at room temperature in an ultrahigh-vacuum magnetron sputtering system onto arrays of cantilevers which had been patterned from 3-in thermally oxidized (1.5 μm SiO 2 ) Si wafers via standard Si bulk micromachining techniques. Each cantilever is 10 mm long, 2 mm wide, and ~70 μm thick. The chamber pressure before deposition was lower than 1×10 −7 Pa, and the Ar pressure during the deposition was 0.6 Pa. To obtain binary composition variation across each wafer, Fe (99.95%) and Co (99.95%) targets were co-sputtered at 60 W and 50 W, respectively. After deposition, the Fe and Co concentration on each cantilever in the spread was mapped by wavelength dispersive X-ray spectroscopy with a JEOL electron probe (JXA-8900R) The compositional variation across each cantilever was less than 1.5 at.%. After the deposition, some of the as-grown spreads were annealed at 800 °C for 1 h in an ultrahigh vacuum chamber with a base pressure lower than 1×10 −9 Pa. Following annealing, the spreads were cooled from high temperature in vacuum either by slow cooling or by quenching. In this study, some spreads were slow-cooled at a rate ~5 °C min −1 , whereas others were water-quenched to room temperature in 1–2 s, yielding a cooling rate of 2.3×10 4 °C min −1 . Cantilever deflection method The magnetostriction of the as-deposited and all annealed composition spread thin film samples were determined using the cantilever deflection method [44] . For this measurement, a 635-nm power-stabilized diode laser (5 mW) was deflected off the tip of each cantilever onto a position sensitive detector ON-TRAK OT301 precision sensing module. Once the magnetic field has been applied, cantilever bending occurs due to the magnetostriction in the film, and the resultant cantilever displacement is captured on the position sensitive detector and measured as a function of the applied field. Careful adjustments were made to ensure that no contribution from torque was included in the displacement output. Displacement measurements were recorded for magnetic fields applied parallel and perpendicular to the length of the cantilever, but always parallel to film plane. The raw parallel ( D ∥ ) and perpendicular ( D ⊥ ) displacements from measurements with two field directions were used to calculate an effective magnetostriction constant ( λ eff ) using the expression of du Tremolet de Lacheisserie and Peuzin [44] : where L is the sample length, E f and E s are Young's moduli of the film and substrate, t f and t s are their respective thicknesses, and v f and v s are their respective Poisson′s ratios. D ∥ and D ⊥ represents the displacement measured when the field is applied along the length and perpendicular to the cantilever, respectively. The λ eff convention used here is convolutions of the cubic constants ( λ 100 and λ 111 ) because the films studied here are either polycrystalline or textured. The films are 0.5 micron thick, and thus, especially in the annealed states, the stress is relaxed and does not affect the measured values of magnetostriction. Determination of the elastic modulus The elastic modulus ( E f ) of the magnetostrictive films at each composition was determined by measuring the change in the resonant frequency of the first flexural mode of each cantilever. The resonant frequency measurements were made with a laser Doppler vibrometer (Polytec MSA-500). The arrays of bare Si cantilevers were measured first, and then re-measured after films were deposited, and again, after they were annealed. This technique is similar to that described by Petersen and Guarnieri [45] . To account for non-uniformities in the cantilever thickness that resulted from the release procedure, the cantilever thickness was back-calculated using Euler–Bernoulli beam theory [46] . From this calculated thickness, the modulus of the deposited films can be determined from equation (4) where E , h , ρ are the modulus, thickness, and density, respectively, with subscripts s and f denoting properties of the substrate and film, respectively. The ratio of the resonance frequencies of the f uni and f bi is not fully simplified to show the full forms of the frequency equations where L is the length of the cantilever and k i is the i th eigenvalue for the flexural mode (3.516 for the first mode). The error represents the 95% confidence intervals for the Lorentzian fit of the resonant peaks at f uni and f bi . Figure 7 shows the dependence of Young's modulus on Co composition for annealed samples. Microstructural characterization The crystal structure of the thin film samples were characterized using synchrotron X-ray microdiffraction at the Stanford Synchrotron Radiation Lightsource (beamline 11-3). Each diffraction measurement was recorded at room-temperature on an image plate detector (MAR 345) with an exposure time of 30 s. The beam size was focused to a 150-μm×150-μm spot, and the photon energy used was 12.7 keV, with the incident angle ( ω ) of the beam set at 5°. The peak positions of the raw data were normalized using NIST LaB 6 standard powder (NIST SRM 660b). d-spacings were extracted from the integrated diffraction rings for each composition. TEM investigations were carried out on a JEOL JEM-3010UHR microscope operated at 300 kV. The magnetic hysteresis loops of the annealed and water-quenched thin film sample were measured using a vibrating sample magnetometer (LakeShore7410 VSM system). How to cite this article: Hunter, D. et al . Giant magnetostriction in annealed Co 1−x Fe x thin-films. Nat. Commun. 2:518 doi: 10.1038/ncomms1529 (2011).